Timing ofSmarcb1andNf2inactivation determines schwannoma versus rhabdoid tumor development Germline mutations of the SMARCB1 gene predispose to two distinct tumor syndromes: rhabdoid tumor predisposition syndrome, with malignant pediatric tumors mostly developing in brain and kidney, and familial schwannomatosis, with adulthood benign tumors involving cranial and peripheral nerves. The mechanisms by which SMARCB1 germline mutations predispose to rhabdoid tumors versus schwannomas are still unknown. Here, to understand the origin of these two types of SMARCB1 -associated tumors, we generated different tissue- and developmental stage-specific conditional knockout mice carrying Smarcb1 and/or Nf2 deletion. Smarcb1 loss in early neural crest was necessary to initiate tumorigenesis in the cranial nerves and meninges with typical histological features and molecular profiles of human rhabdoid tumors. By inducing Smarcb1 loss at later developmental stage in the Schwann cell lineage, in addition to biallelic Nf2 gene inactivation, we generated the first mouse model developing schwannomas with the same underlying gene mutations found in schwannomatosis patients. Germline alterations of SMARCB1 gene predispose to two different inherited tumor syndromes: rhabdoid tumor predisposition syndrome (MIM 609322) [1] and familial schwannomatosis (MIM 162091) [2] . The first genetic evidence of the role of SMARCB1 as a tumor suppressor was the identification of its biallelic mutations as the cause of most cases of malignant rhabdoid tumors (RTs) [3] , [4] , a highly aggressive pediatric cancer that usually occurs in the brain (named atypical teratoid rhabdoid tumor: AT/RT), kidneys and soft tissues in the first years of life. Heterozygous SMARCB1 mutations are the basis of the rhabdoid tumor predisposition syndrome [3] , [5] . More recently, SMARCB1 has been identified as a predisposing gene in familial schwannomatosis [6] , a condition characterized by the onset of multiple spinal, peripheral, and cranial-nerve schwannomas during adulthood in the absence of vestibular schwannomas [7] . Five percent of schwannomatosis patients also develop cranial or spinal meningiomas [8] . SMARCB1 germline mutations have been found in 45% of familial probands and 7% of sporadic schwannomatosis patients [9] . Although the exact molecular pathogenetic mechanisms in these schwannomas remain to be elucidated, a 4-hit/3-step mechanism involving SMARCB1 and NF2 genes seems to underlie development of these benign tumors in schwannomatosis patients [10] . Germline mutations in LZTR1 , a gene closely linked to NF2 and SMARCB1 on chromosome 22, have recently been identified in a significant proportion of schwannomatosis patients lacking SMARCB1 germline mutations. Similar to SMARCB1 -related schwannomas, different additional somatic mutations in NF2 were identified in schwannomas from these patients, thus supporting the 4-hit/3-step hypothesis [11] . This mechanism reinstates the crucial role of biallelic NF2 loss in schwannoma genesis and of developmental risk periods for SMARCB1 and NF2 mutations to occur. In contrast, a single case of double SMARCB1/NF2 inactivation was found in RTs [12] . Recent analysis of a larger series confirmed SMARCB1 as the primary tumor suppressor gene involved in the development of rhabdoid tumors with no recurrent additional oncogenic canonical pathway mutations identified [13] . This raises challenging questions about the molecular mechanisms by which germline mutations in the same gene predispose to early aggressive RTs versus late-onset benign PNS tumors. Analysis of the SMARCB1 gene mutation spectrum points to genotype-phenotype correlations, with germline rhabdoid tumor mutations being more centrally placed in the coding sequence, involving multiple exons and truncating mutations of the SMARCB1 gene. Conversely, schwannomatosis mutations are mostly non truncating mutations and located in hot spots at both 5′ and 3′ end of the SMARCB1 gene [14] . However, families with RTs or multiple epitheloid schwannomas sharing the same SMARCB1 mutation have also been described [15] , [16] , [17] . A link between schwannoma and RT has also been suggested by the histological analysis of a series of aggressive PNS tumors revealing rhabdoid features [18] , [19] , [20] , and sporadic case reports of RTs emanating from cranial nerves [21] , [22] , [23] . Altogether, these observations raise the question of whether the two types of SMARCB1 -deficient tumors arise from common or different progenitor cells. In mice, the specific deletion of the Nf2 gene in P0 permissive cells targets the cells of origin of schwannomas in cranial nerves, peripheral nerves, and nerve roots [24] , [25] . Although different hypotheses have been suggested, the cell of origin of RTs remains unclear. Different studies using histological and molecular markers or mouse models suggested that RTs could arise from the mesenchymal lineage [26] , neural progenitor cells [27] , neural crest stem cells [28] , [29] , [30] , [31] , stem cells [32] , germ and/or embryonic stem cells [33] . The homozygous inactivation of Smarcb1 in mice leads to peri-implantation lethality and heterozygous mice develop RTs at low penetrance (15–30%) [29] , [31] , [34] . In two different Smarcb1 +/− mouse models, RTs developed predominantly in the soft tissues of the head and neck [29] , [34] . In another Smarcb1 +/− model, 30% of the mice developed intra-cranial tumors and 27% in the spinal cord around the dorsal ganglia or spinal nerves that were classified as undifferentiated sarcomas with variable rhabdoid features [31] . All three types of Smarcb1 +/− mice presented an extended time window for tumor onset with the earlier appearance at 3–4 months of age and median onset at 11–12 months of age, depending on the model [29] , [31] , [34] . Conditional Smarcb1 inactivation in all tissues except the brain led to 100% of mice developing T-cell lymphoma with 13% of mice developing RTs with a median latency of 11 weeks after induction, demonstrating that inactivation of the second Smarcb1 allele is rate limiting RT development in Smarcb1 +/− mice [35] . To investigate the role of Smarcb1 loss in PNS tumorigenesis, we conditionally inactivated Smarcb1 in neural crest (NC) and Schwann cell (SC) lineages. We report that tumors arising from neural crest cells (NCCs) have histological and molecular characteristics of human RTs, providing novel clues to their cellular origin. Finally, we show that biallelic inactivation of Smarcb1 and Nf2 in SCs results in benign schwannoma, and not in RT, thus re-emphasizing the necessary and sufficient role of NF2 loss in SC tumorigenesis, in both neurofibromatosis type 2 (NF2) and schwannomatosis, and the existence of a critical developmental risk period for SMARCB1 -deficient RTs to occur. Smarcb1 loss in early NC promotes RT development We tested the hypothesis that Smarcb1 inactivation in NCCs and in the SC lineage is sufficient to initiate schwannoma development in the mouse. Fifty percent of mice (3/6) carrying a germline Smarcb1 deleted allele ( Smarcb1 del/+ ) developed tumors with rhabdoid features occurring over a wide age range (2–17 months of age). This observation is in line with the tumor phenotype described in other mouse models of Smarcb1 inactivation [29] , [31] , [34] . Tumors were located in the brain (emergence of trigeminal nerve), spinal nerve roots and on the cheek and did not present histological features of schwannoma. To circumvent the early lethality of Smarcb1 −/− mutants and malignant tumors found in Smarcb1 del/+ mice, we used a conditional floxed Smarcb1 allele ( Smarcb1 flox ) [36] . To define the temporal window of susceptibility to Smarcb1 loss, we used different promoters to induce Cre-mediated Smarcb1 deletion at different stages of SC development. To specifically direct Cre recombinase expression to the NCCs at E9.5 and SC lineage we chose the promoter of the protein zero (P0) gene, which efficiently targets schwannoma precursor cells [24] , [25] . P0-CreC;Smarcb1 flox/flox mice, harboring a homozygous deletion of Smarcb1 , were viable and obtained at the expected Mendelian ratio (21.6 vs. 25%, non-statistically significant difference, Fig. 1a ). Fig. 1 P0-CreC;Smarcb1 flox/flox mice develop RTs in NC-derived tissues. a Genotype distribution of mice at 3 weeks of age ( n = 282) born from crossings of P0-CreC;Smarcb1 flox/+ and Smarcb1 flox/flox mice. b Kaplan–Meier curve representing the percent survival of P0-CreC;Smarcb1 flox/flox ( n = 141, median survival = 3.2 months), P0-CreC;Smarcb1 flox/+ ( n = 29, median survival = 21.6 months) and Smarcb1 flox/flox ( n = 33, median survival > 24 months) mice versus age in months. c T2-weighted MR image identifying a tumor mass in the nasal cavities of a P0-CreC;Smarcb1 flox/flox mouse ( arrow ). d X-gal staining of a tumor from P0-CreC;Smarcb1 flox/flox ; ACZL mice demonstrating activation of the beta-galactosidase reporter gene ACZL ( blue staining) thus attesting for Smarcb1 deletion throughout the tumor and in rhabdoid cells ( arrow and inset ). e Smarcb1 del allele is detected in all the tumors from young P0-CreC;Smarcb1 flox/flox mice (< 10 months of age). Long-term P0-CreC;Smarcb1 flox/flox survivor mice (Supplementary Fig. 2c ) develop liver, lung, and uterus tumors, with no deletion of Smarcb1 similar to control littermates ( Smarcb1 flox/flox ). These tumors are part of the normal tumor spectrum of aging FVB/N mice [24] . f , g P0-CreC;Smarcb1 flox/flox mice develop tumors along the olfactory nerve ( arrow ), close to the olfactory bulb ( f ) or in the nasal cavity below the olfactory epithelium ( double arrow , g ). h X-gal staining of the nasal cavity of a P0-CreC;AZCL mouse showing specific Cre recombinase expression in SCs of the olfactory nerve ( arrow ) below the olfactory epithelium layer ( double arrow ). i Tumor of the trigeminal nerve (transversal section). j X-gal staining of the trigeminal nerve of a P0-CreC;AZCL mouse showing specific Cre recombinase expression in SCs (arrows). k Tumor of the vestibulocochlear nerve ( dashed square ) invading the cochlea ( arrow ). Note that the contralateral side is not affected. l Detail of the vestibulocochlear nerve tumor shown in k . m Tumors in the eye ( black arrow ), optic nerve ( white arrow ), and oculomotor nerve ( striped arrow ) of a P0-CreC;Smarcb1 flox/flox mouse. n Tumors in the spinal nerve roots ( arrows , longitudinal section). Insets in f , i , l , m and n represent a higher magnification of the dashed square area ( insets scale bar is 20 µm). **( P < 0.01) and ***( P < 0.001); log-rank (Mantel–Cox) test Full size image P0-CreC;Smarcb1 flox/flox mice presented with mild craniofacial abnormalities: orbit malformations and misshapen mandibles, with dental malocclusion eventually leading to outgrowing teeth. Few mice displayed bloated intestines with histological analysis revealing emaciated intestine wall associated with a reduced number of villi. About 65% of P0-CreC;Smarcb1 flox/flox mice developed tumors between 1.5 and 5 months of age with an overall median survival of 3.2 months (Fig. 1b ). These mice developed aggressive cranial nerve tumors: olfactory (91%, Fig. 1c, f, g ), trigeminal (51%, Fig. 1i ), oculomotor and optic (37%, Fig. 1m ), or vestibulocochlear (14%, Fig. 1k, l ) nerves were the most affected. Tumors were also found in the meninges with variable extent of brain invasion (14%, Fig. 2a, b ), in spinal nerve roots (3%, Fig. 1n ) and occasionally in the eye (Fig. 1m ), with 62.5% (15/24) of the mice displaying multiple tumors at dissection. In all mice presenting with a head tilt and/or spinning behavior, unilateral tumors of the vestibular nerve ganglion and/or invasion of the inner ear were found (Fig. 1k, l ). Use of the P0-CreB transgenic mice, which express Cre recombinase at E9.5, similarly to P0-CreC , but in a larger number of cells [25] , resulted in a more severe phenotype with a lower percentage of viable P0-CreB;Smarcb1 flox/flox mice (1.4 vs. 25% expected, P < 0.0001, Supplementary Fig. 1a ). Nasal cavity or retro-orbital tumors, with the same histological features than P0-CreC;Smarcb1 flox/flox tumors were found in 62.5% of P0-CreB;Smarcb1 flox/flox mice between 1.2 and 2 months of age (Supplementary Fig. 1b ). Tumor location in P0-CreC;Smarcb1 flox/flox mice correlated with the expression pattern of the P0-CreC transgene (Supplementary Fig. 2a ). X-gal staining of olfactory epithelium (Fig. 1h ) and trigeminal nerve (Fig. 1j ) in P0-CreC;ACZL mice [25] demonstrated the presence of Cre activity in few cells that are likely the cells of origin of tumors in P0-CreC;Smarcb1 flox/flox mice. Tumors developed by P0-CreC;Smarcb1 flox/flox ; ACZL mice before 10 months of age displayed a blue X-gal staining, demonstrating the Cre recombinase activity and Smarcb1 deletion, including in rhabdoid cells (Fig. 1d ). The presence of the Smarcb1 deleted allele in all tumors from symptomatic P0-CreC;Smarcb1 flox/flox mice was confirmed by PCR analysis (Fig. 1e ). Despite expression of the Cre recombinase and detection of the Smarcb1 deleted allele, tumors were not found in kidneys, gonads and in brachial, saphenous and sciatic nerves of P0-CreC ; Smarcb1 flox/+ and P0-CreC;Smarcb1 flox/flox mice (Supplementary Fig. 2a, b ). This finding can be explained either by the fact that Cre in P0-CreC and P0-CreB mice is not expressed in the cell of origin of kidney RTs, or is not expressed during the specific temporal window of vulnerability to RT development. No pathological alteration was found in nerves (cranial, phrenic, saphenous, sciatic nerves, and brachial plexus), DRGs and brain in long-term P0-CreC;Smarcb1 flox/flox survivor mice (up to 24 months of age). Fig. 2 P0-CreC;Smarcb1 flox/flox mice develop RTs in the meninges. a Supratentorial tumors ( white arrow ) were found predominantly located in the subarachnoid space ( black arrow, inset ) with extension into the brain parenchyma. Inset represents a higher magnification of the dashed square area . b Detail of a tumor originating from the meninges. The arrow shows the arachnoid cell layer. c No PGDS staining was found in the tumor as opposed to the arachnoid cell layer ( arrow ). d , e The GFAP staining demonstrated the different degree ( d , non-invasive; e , irregular tumor brain interface consistent with infiltration) of invasiveness of the tumors in the brain tissue Full size image P0-CreC;Smarcb1 flox/flox tumors display human RT features Tumors of P0-CreC;Smarcb1 flox/flox mice displayed a histologic spectrum ranging from a primitive neuroectodermal (Fig. 3a ), to a mesenchymal (Fig. 3b ) or rhabdoid pattern (Fig. 3c ). No epithelial differentiation was observed. Most tumor cells exhibited atypical large nuclei with vesicular chromatin, irregular and thick membrane, and prominent nucleoli (Fig. 3b inset ). Some of these cells showed an eccentric nucleus associated with a prominent eosinophilic cytoplasmic inclusion (Fig. 3c and inset ) or cytoplasmic vacuolar degeneration (Fig. 3d and inset ), typical histological features encountered in human AT/RTs [37] . Rhabdoid features or scattered rhabdoid cells were found in all analyzed tumors, and in 30% of these, nests of rhabdoid cells were present (Fig. 3c ). Bi-nucleated and giant multinucleated cells were also found in some tumors. Tumors displayed different patterns depending on their size at the time of dissection. Larger tumors typically presented more rhabdoid features than smaller tumors. All the tumors examined demonstrated loss of SMARCB1 nuclear expression by immunohistochemical staining (Fig. 3e ). However, similar to human RTs [38] , infiltrating inflammatory and endothelial cells retained SMARCB1 staining (Fig. 3e ). The tumors behaved in an aggressive manner, displaying rapid growth, moderate to high cellularity and abundant mitotic figures with high percentages of Ki-67-positive cells (50.7 ± 3.7% in neuroectodermal and 33.4 ± 3.9% in mesenchymal histological subtypes) (Fig. 3f ). Larger tumors frequently showed areas of necrosis. Some tumors were contained within the boundaries of the tissue of origin, such as the epineurium of the trigeminal nerve (Fig. 1i ), while other tumors, such as those extending in the cochlea from the vestibulocochlear nerve, were more invasive, (Fig. 1k, l ). Supratentorial rhabdoid tumors were found predominantly located in the subarachnoid space with extension into the brain parenchyma (Fig. 2a, b ). These tumors displayed well-demarcated smooth borders with adjacent tissues and reactive gliosis confirmed with GFAP staining in adjacent tissues to the tumor (Fig. 2d ). In some cases, individual tumor cells were invading the brain parenchyma (Fig. 2e ). The location of these tumors suggested that they originated outside of the brain parenchyma and developed from the cranial NC-derived meningeal progenitor cells [39] . The absence of PGDS staining (Fig. 2c ), an arachnoid cell marker expressed postnatally in the NC-derived meninges, substantiates the hypothesis that meningeal RTs originate from early NC-derived progenitor cells, before differentiation in PGDS-positive arachnoid cells [39] . Fig. 3 RTs of P0-CreC;Smarcb1 flox/flox mice display typical histological and immunohistochemical staining features of human RTs. a Tumor presenting a primitive neuroectodermal pattern. b Tumor with mesenchymal pattern characterized by spindle-shaped cell component and nuclei showing vesicular chromatin staining pattern with prominent nucleoli ( arrows and inset ). c Nest of classic rhabdoid cells with eccentrically placed nuclei, vesicular chromatic staining and eosinophilic cytoplasm inclusion ( arrows and inset ). d Tumor demonstrating vacuolar cytoplasmic degeneration pattern ( arrow and inset ). e SMARCB1 staining shows loss of nuclear expression in tumor cells with retained expression in infiltrating inflammatory cells and intratumoral vasculature ( arrow ). f Ki-67 staining reveals high proliferative index. g Diffuse strong expression of vimentin in tumor tissue from P0-CreC;Smarcb1 flox/flox mice. Note the staining of the cytoplasmic inclusions in rhabdoid cells ( arrow and inset ). h Foci of tumors cells show positive cytoplasmic staining for SMA. i , j No staining of cytokeratins i and neurofilament triplet proteins j were found in the tumors. k Strong S100 immunoreactivity in schwannoma from P0-CreC;Nf2 flox/flox mice. l No S100 staining is present in the tumors cells of P0-CreC;Smarcb1 flox/flox mice. Sparse positive cells are entrapped residual normal cells. m Moderate GFAP staining in P0-CreC;Nf2 flox/flox schwannoma. n No GFAP staining is present in the tumors cells of P0-CreC;Smarcb1 flox/flox mice. o , p Strong expression of FABP7, an early marker of SC precursors, in P0-CreC;Nf2 flox/flox o and P0-CreC;Smarcb1 flox/flox p tumors. Scale bars : 50 µm for main pictures and 10 µm for insets Full size image Because of their heterogeneous histologic features, RTs usually show a broad spectrum of immunohistochemical reactivity [40] . With a remarkable similarity to human RTs [37] , tumors from P0-CreC;Smarcb1 flox/flox mice typically showed a consistent expression of vimentin (Fig. 3g ), a moderate to strong SMA staining (Fig. 3h ), whereas staining for cytokeratin proteins or neurofilament triplet proteins, commonly found in foci of human AT/RTs, was not detected (Fig. 3i, j ). Staining of S100 protein, a marker of schwannoma [41] , allowed to clearly distinguish the P0-CreC;Smarcb1 flox/flox mouse tumors from schwannomas: unlike schwannomas from P0-CreC;Nf2 flox/flox mice, which strongly and diffusely express S100 protein (Fig. 3k ), tumor cells from P0-CreC;Smarcb1 flox/flox mice showed no S100 protein by IHC (Fig. 3l ). Modest GFAP expression was present in P0-CreC;Nf2 flox/flox tumors (Fig. 3m ) whereas P0-CreC;Smarcb1 flox/flox tumors showed little GFAP expression in few reactive astrocytes (Fig. 3n ). However, tumors from both P0-CreC;Smarcb1 flox/flox and P0-CreC;Nf2 flox/flox mice displayed a strong staining for FABP7 (Fatty Acid Binding Protein 7) (Fig. 3o, p ), an early marker of SC precursors [42] . Altogether, P0-CreC;Smarcb1 flox/flox mouse tumors displayed typical histological and immunohistochemical features of human RTs, clearly distinguishable from Nf2 -deficient P0-CreC;Nf2 flox/flox schwannomas (Fig. 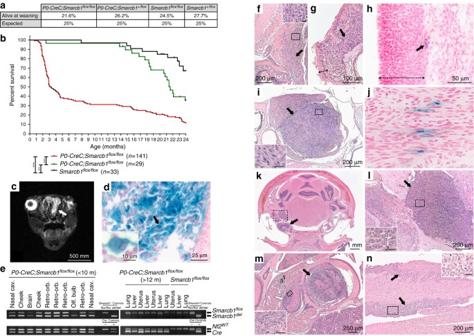Fig. 1 P0-CreC;Smarcb1flox/floxmice develop RTs in NC-derived tissues.aGenotype distribution of mice at 3 weeks of age (n= 282) born from crossings ofP0-CreC;Smarcb1flox/+andSmarcb1flox/floxmice.bKaplan–Meier curve representing the percent survival ofP0-CreC;Smarcb1flox/flox(n= 141, median survival = 3.2 months),P0-CreC;Smarcb1flox/+(n= 29, median survival = 21.6 months) andSmarcb1flox/flox(n= 33, median survival > 24 months) mice versus age in months.cT2-weighted MR image identifying a tumor mass in the nasal cavities of aP0-CreC;Smarcb1flox/floxmouse (arrow).dX-gal staining of a tumor fromP0-CreC;Smarcb1flox/flox;ACZLmice demonstrating activation of the beta-galactosidase reporter geneACZL(bluestaining) thus attesting forSmarcb1deletion throughout the tumor and in rhabdoid cells (arrow and inset).eSmarcb1delallele is detected in all the tumors from youngP0-CreC;Smarcb1flox/floxmice (< 10 months of age). Long-termP0-CreC;Smarcb1flox/floxsurvivor mice (Supplementary Fig.2c) develop liver, lung, and uterus tumors, with no deletion ofSmarcb1similar to control littermates (Smarcb1flox/flox). These tumors are part of the normal tumor spectrum of aging FVB/N mice24.f,gP0-CreC;Smarcb1flox/floxmice develop tumors along the olfactory nerve (arrow), close to the olfactory bulb (f) or in the nasal cavity below the olfactory epithelium (double arrow,g).hX-gal staining of the nasal cavity of aP0-CreC;AZCLmouse showing specificCrerecombinase expression in SCs of the olfactory nerve (arrow) below the olfactory epithelium layer (double arrow).iTumor of the trigeminal nerve (transversal section).jX-gal staining of the trigeminal nerve of aP0-CreC;AZCLmouse showing specificCrerecombinase expression in SCs (arrows).kTumor of the vestibulocochlear nerve (dashed square) invading the cochlea (arrow). Note that the contralateral side is not affected.lDetail of the vestibulocochlear nerve tumor shown ink.mTumors in the eye (black arrow), optic nerve (white arrow), and oculomotor nerve (striped arrow) of aP0-CreC;Smarcb1flox/floxmouse.nTumors in the spinal nerve roots (arrows, longitudinal section).Insetsinf,i,l,mandnrepresent a higher magnification of thedashed square area(insets scale baris 20 µm). **(P< 0.01) and ***(P< 0.001); log-rank (Mantel–Cox) test 3 and Supplementary Table 1 ) [37] . Molecular profiling classifies mouse RTs in three subgroups To address the relevance of the P0-CreC;Smarcb1 flox/flox mouse tumors as models of the human condition, we profiled 12 representative RTs by whole-genome RNA sequencing. Unsupervised hierarchical clustering of the top 5000 most variable transcripts in P0-CreC;Smarcb1 flox/flox RTs identified three molecular subgroups (Supplementary Fig. 3a ). Based on the maximum cophenetic correlation score (non-negative matrix factorization (NMF) method), the optimal number of clusters was estimated to be two or three (Supplementary Fig. 3b, c ). Across species unsupervised cluster analysis of the top 5000 most variable transcripts in P0-CreC;Smarcb1 flox/flox and human RTs from Johann et al., showed that mouse tumors distributed among the three recently identified human AT/RT molecular subgroups [43] , independent of their anatomical origin (Fig. 4a ). Thus, tumors from P0-CreC;Smarcb1 flox/flox mice recapitulate the molecular diversity of human AT/RTs. According to their inclusion in different human AT/RT clusters, we attributed similar molecular subgroups to the P0-CreC;Smarcb1 flox/flox RTs (mRT-Myc, mRT-Shh or mRT-Tyr). In a unsupervised cluster analysis of gene expression profiles from P0-CreC;Smarcb1 flox/flox , Rosa26-Cre ERT2 ;Smarcb1 flox/flox [30] and hGFAP-Cre;Smarcb1 flox/flox ;Trp53 flox/flox [44] RT mouse models, tumors segregated based on molecular subgroups rather than on the model of origin, demonstrating their molecular analogy (Fig. 4b ). We conducted Weighted Gene Co-expression Network Analysis (WGCNA), a systems biology approach used to identify networks of co-expressed genes in relation to phenotypic data, using the R package. WGCNA allowed identification, within the highest positively correlated module with each molecular subgroup, of several representative marker genes that were significantly and consistently overexpressed in both human and mouse RT molecular subgroups (Fig. 4c ). Specifically, TRPM3 (Transient Receptor Potential cation channel subfamily M member 3), a membrane channel that can promote renal cell tumors [45] , was found consistently overexpressed in the human hTYR and mouse mRT-Tyr molecular subgroups (Fig. 4c ). HDGFRP3 (Hepatoma-Derived Growth Factor, Related Protein 3), which plays an essential role in hepatocellular carcinoma pathogenesis [46] and LOXL4 (Lysyl Oxidase Like 4), which promotes proliferation and metastasis of gastric cancer [47] , were consistently overexpressed in mouse and human SHH and MYC molecular subgroups, respectively (Fig. 4c ). TYR , MYCN , and HOTAIR , marker genes of the three human subgroups [43] showed a similar trend of overexpression in the respective mouse RT subgroups, albeit not statistically significant likely due to the small number of mouse tumors analyzed (Fig. 4c ). Fig. 4 Molecular profiling of RTs from P0-CreC;Smarcb1 flox/flox mice. a Unsupervised hierarchical clustering of gene expression profiles from 12 P0-CreC;Smarcb1 flox/flox mouse tumors and 49 human AT/RTs [43] using the 5,000 most variable transcripts. The P0-CreC;Smarcb1 flox/flox tumors distributed among the three human AT/RT molecular subgroups. Information about tumor molecular subgroups and anatomical location is displayed in the lower bars. b Unsupervised hierarchical clustering of gene expression profiles from 12 P0-CreC;Smarcb1 flox/flox mouse tumors, eight tumors from the tamoxifen inducible Rosa26-Cre ERT2 ;Smarcb1 flox/flox mouse model [30] and five tumors from the hGFAP-Cre;Smarcb1 flox/flox ;Trp53 flox/flox mouse model [44] using the 5,000 most differentially expressed genes. Information about tumor molecular subgroups is displayed in the lower bars. c Normalized expression level of representative genes for both of the three human AT/RT molecular subgroups: hTYR ( n = 16), hSHH ( n = 16), and hMYC ( n = 17) and the three P0-CreC;Smarcb1 flox/flox RT molecular subgroups: mRT-Tyr ( n = 5), mRT-Shh ( n = 4) and mRT-Myc ( n = 3). On the basis of the cluster analysis in ( a ), we respectively named hMYC, hSHH and hTYR the three tumor subgroups including human tumors from the MYC, SHH and TYR molecular subgroups [43] . The P -value indicates the statistical significance of gene enrichment within their respective WGCNA module for each respective molecular subgroup. d – g Gene expression levels of specific SWI/SNF complex subunits ( d , e ) and NC developmental markers ( f , g ) in the three molecular subgroups of P0-CreC;Smarcb1 flox/flox RTs ( d , f ) and human AT/RTs ( e , g ). d , f RNA-Seq data are expressed in RPKM (Reads Per Kilobase of transcript per Million mapped reads). e , g graphs of microarray gene-expression intensity from dataset GSE70678. c – g RNA-Seq and microarray gene expression levels are shown using Tukey boxplots: the central lines represent the median, boxes (interquartile range or IQR) represent 50% of data ranging from the 25 to 75% quantile, whiskers represent extremes up to 1.5-fold box size, circles show outliers Full size image As in human AT/RTs [48] , Smarcb1 deficiency in all P0-CreC;Smarcb1 flox/flox RT subgroups was correlated with an increased expression of the polycomb gene Ezh2 (Supplementary Fig. 4a, b ), a key driver of oncogenesis [49] . Analysis of molecular pathways in P0-CreC;Smarcb1 flox/flox RTs by western blot showed increased phosphorylation of Akt, S6, and 4E-BP1, consistent with activation of the mTOR/Akt pathway, similar to schwannomas in P0-CreC;Nf2 flox/flox mice (Supplementary Fig. 4c ). Cell cycle proteins (CDK4, CDK6, cyclin D1, p16) were overexpressed in all P0-CreC;Smarcb1 flox/flox tumors and phosphorylation of the retinoblastoma protein was found in 3 out of 5 RTs (Supplementary Fig. 4c ). Activation of these pathways has been reported in human RTs [50] . Early NC molecular signature in Smarcb1 -deficient RTs To explore the effect of Smarcb1 deficiency on the SWI/SNF complex in P0-CreC;Smarcb1 flox/flox mouse RTs, we analyzed the expression of the different complex subunits using the RNA-Seq gene expression data. High expression of Actl6a (BAF53a), Phf10 (BAF45a), Dpf2 (BAF45d), and Ss18 (SYT) genes, encoding subunits found in the pluripotent embryonic stem cell (esBAF) and in the multipotent neural progenitor (npBAF) complexes [51] was found in RTs of all three molecular subgroups (Fig. 4d ). In contrast, mouse RTs did not express Actl6b (BAF43b), Dpf1 (BAF45b), Dpf3 (BAF45c) and Ss18l1 (CREST) genes, encoding subunits exclusively found in the postmitotic neural BAF complex (nBAF) (Fig. 4d ). These results, except for SS18L1 (CREST), were consistent with subunit gene expression in the series of human AT/RTs from Johann et al . (Fig. 4e ) and demonstrated that the residual SWI/SNF complex in Smarcb1 -deficient RTs is characteristic of undifferentiated progenitor cells [51] , pointing to an early developmental cell population of origin for RTs. Analysis of gene regulatory networks underlying formation of NCCs showed robust expression of genes exclusively expressed in the neural plate border and NC specification modules [52] in both P0-CreC;Smarcb1 flox/flox and human RT samples (Fig. 4f, g ). The fact that human AT/RTs and RTs from P0-CreC;Smarcb1 flox/flox mice retain specific marker genes of early NC formation, strongly corroborates the hypothesis of an early NCC as their cell of origin. SC differentiation suppresses Smarcb1 -driven tumorigenicity The existence of adult carriers of a SMARCB1 mutation without RT in families presenting either RTs or schwannomas suggests the existence of a specific developmental time window during which RT progenitor cells are vulnerable to SMARCB1 loss [15] , [16] , [17] . To assess if loss of Smarcb1 at a later stage of development would induce tumorigenesis, we bred Smarcb1 flox mice with DHH-Cre and mGFAP-Cre transgenic mice that express the Cre recombinase at later stages of SC development. DHH-Cre transgenic mice [53] express Cre in SC precursors beginning at embryonic day E12.5 [42] . DHH-Cre;Smarcb1 flox/flox mice had an overall median survival of 3 weeks and displayed progressive hindlimb paralysis. The sciatic nerves were thinner and more transparent than in control littermates. Histological analysis demonstrated that loss of Smarcb1 (Supplementary Fig. 5c, d ) led to a lack of structure and organization of the nerve fibers (Supplementary Fig. 5a, b ) with increased numbers of BrdU and Ki-67 positive cells (Supplementary Fig. 5e–h ). No tumors were found in cranial nerves, peripheral nerves, or dorsal root ganglions (DRGs) of DHH-Cre;Smarcb1 flox/flox mice during their short lifespan. To target immature SCs, we generated mGFAP-Cre;Smarcb1 flox/flox mice using the mGFAP-Cre transgenic mice that express the Cre recombinase under the promoter of the mouse GFAP gene [54] . This promoter targets immature SCs in the peripheral nervous system starting at E13.5 [54] , postnatal astrocytes throughout the CNS and postnatal astroglial cells in the cerebellum [55] . X-gal staining of tissues from mGFAP-Cre;ACZL mice demonstrated expression of Cre recombinase in spinal nerve root SCs (Supplementary Fig. 6d ), spinal cord and throughout the brain (Supplementary Fig. 6c ). At three months of age, mGFAP-Cre;Smarcb1 flox/flox and mGFAP-Cre;Smarcb1 del/flox mice started developing cataracts, displayed progressive ataxia with loss of motor coordination and gait balance, eventually leading to loss of bodyweight and euthanasia. This neurological phenotype was similar to the one described at earlier age in hGFAP-Cre;Smarcb1 flox/flox [56] and hGFAP-Cre;Smarcb1 flox/flox ;Trp53 flox/flox [44] mice. The median survival of mGFAP-Cre;Smarcb1 flox/flox and mGFAP-Cre;Smarcb1 del/flox mice was 3.7 and 3.8 months of age ( P = 0.74, non-statistically significant difference, Supplementary Fig. 6b ), respectively. Histological analysis of the brain revealed atrophy of the cerebellum, but no tumors were found in the brain, cranial nerves or DRGs (Supplementary Fig. 6e, f ). No change in cellularity was found in the DRGs of mGFAP-Cre;Smarcb1 flox/flox mice compared with control littermates (Fig. 5a, b, g ). Fig. 5 Biallelic loss of Nf2 is necessary to induce schwannoma formation. a , b No difference in cellularity of DRGs from mGFAP-Cre;Smarcb1 flox/flox mice ( b ) compared with Smarcb1 flox/flox control mice ( a ). c – f The loss of one additional Nf2 allele in mGFAP-Cre;Smarcb1 flox/flox ;Nf2 flox/+ mice does not impair the DRG cellularity ( d ) compared to mGFAP-Cre;Smarcb1 flox/flox mice ( b ) or Smarcb1 flox/flox ;Nf2 flox/flox control mice ( c ). The biallelic loss Nf2 induced the formation of schwannoma tumorlets in mGFAP-Cre;Smarcb1 flox/flox ;Nf2 flox/flox mice ( e ), similar to mGFAP-Cre;Nf2 flox/flox mice ( f ). g Number of cells per DRG surface for each genotype. Data are represented as mean ± s.e.m. ; n is the number of DRG analyzed per genotype, ns (not significant), ***( P < 0.001), two-tailed unpaired Student’s t -test Full size image In conclusion, the observation that DHH-Cre;Smarcb1 flox/flox and mGFAP-Cre;Smarcb1 flox/flox mice did not develop RTs allowed us to narrow down to early NC development the time window for Smarcb1 loss to promote malignant tumorigenesis. Smarcb1 and Nf2 loss in SCs promotes schwannoma development The observation of frequent somatic, tumor-specific NF2 mutations, and the loss of the second NF2 allele in schwannomas from patients with germline SMARCB1 mutations [10] , [57] , [58] , [59] strongly suggest that the classical two-hit model of tumorigenesis does not pertain in the tumors of schwannomatosis patients, as it would require biallelic SMARCB1 inactivation to be sufficient for tumor initiation or growth [7] . Thus, we tested the hypothesis that NF2 loss is necessary for schwannoma formation in schwannomatosis patients with germline SMARCB1 mutations. To model the different steps leading to the double SMARCB1 / NF2 gene loss, we generated combinatorial Smarcb1 and Nf2 wild-type or mutant alleles, representative of the 4-hit/3-step model. P0-CreC;Smarcb1 flox/flox ;Nf2 flox/flox mice were not viable, demonstrating that loss of both Smarcb1 and Nf2 during early development is lethal. However, in mGFAP-Cre;Smarcb1 flox/flox ;Nf2 flox/flox mice, combination of Smarcb1 and Nf2 inactivation resulted in viable mice, with a median survival of 6.4 months of age. The statistically significant longer survival is due to the fact that these mice do not develop the rapidly growing RTs inevitably causing death in P0-CreC;Smarcb1 flox/flox mice. Cre is expressed in the DRGs of mGFAP-Cre mice starting at E13.5 [54] . The mGFAP-Cre;Smarcb1 flox/flox ;Nf2 flox/flox mice developed tumorlets consisting of whorls of SCs in the DRGs (Fig. 5e ). These DRG lesions are similar to those described in the P0-CreC;Nf2 flox/flox [25] and mGFAP-Cre;Nf2 flox/flox mice, and are reminiscent of the schwannoma tumorlets found in NF2 patients [60] , thus demonstrating the necessary role of Nf2 loss for schwannoma formation. Schwannoma tumorlets in the DRGs of mGFAP-Cre;Smarcb1 flox/flox ;Nf2 flox/flox mice were negative for SMARCB1 and merlin staining, about 60% were positive for S100 protein staining, and all were positive for GFAP and FABP7 (Fig. 6 ). The mGFAP-Cre;Smarcb1 flox/flox ;Nf2 flox/+ mice showed similar phenotype to mGFAP-Cre; Smarcb1 flox/flox ;Nf2 flox/flox mice (cataracts, impaired motor coordination and gait balance), leading to a median survival of 7.1 months of age. Similarly to mGFAP-Cre;Smarcb1 flox/flox mice, the decreased and altered mobility of mGFAP-Cre;Smarcb1 flox/flox ;Nf2 flox/flox and mGFAP-Cre;Smarcb1 flox/flox ;Nf2 flox/+ mice led to bodyweight loss and euthanasia. Interestingly, no schwannoma tumorlets were found in the DRGs of mGFAP-Cre;Smarcb1 flox/flox ;Nf2 flox/+ mice, which contained similar cellularity as DRGs of Smarcb1 flox/flox ;Nf2 flox/flox control mice (0.0028 vs. 0.0028 cells/µm 2 , P = 0.94) (Fig. 5c, d, g ) and mGFAP-Cre;Smarcb1 flox/flox mice (0.0028 vs. 0.0026 cells/µm 2 , P = 0.35) (Fig. 5b, d, g ). However, DRGs of mGFAP-Cre;Smarcb1 flox/flox ;Nf2 flox/flox mice showed a significantly increased cellularity compared to those of mGFAP-Cre;Smarcb1 flox/flox ;Nf2 flox/+ mice (0.0044 vs. 0.0028 cells/µm 2 , P = 0.0008) (Fig. 5d, e, g ), thus demonstrating the crucial and necessary role of biallelic Nf2 loss for schwannoma formation. Ki-67 staining identified the presence of few proliferating cells in the DRGs, including in the mGFAP-Cre;Smarcb1 flox/flox ;Nf2 flox/flox and mGFAP-Cre;Nf2 flox/flox schwannoma tumorlets (Fig. 6 ). Surprisingly, complete loss of Smarcb1 in the mGFAP-Cre;Smarcb1 flox/flox ;Nf2 flox/flox tumors did not result in increased cell proliferation compared to schwannoma tumorlets in DRGs from mGFAP-Cre;Nf2 flox/flox mice (Fig. 5f, g ). The very low percentage of proliferating cells in the DRGs of mGFAP-Cre;Smarcb1 flox/flox ;Nf2 flox/flox mice reflects the benign nature of these tumors compared with malignant RTs in P0-CreC;Smarcb1 flox/flox mice (Figs. 3 , 5 and 6 ). Fig. 6 Histological characterization of DRGs and schwannoma tumorlets in control, mGFAP-Cre;Smarcb1 flox/flox , mGFAP-Cre;Smarcb1 flox/flox ;Nf2 flox/flox , and mGFAP-Cre;Nf2 flox/flox mice. DRGs from mGFAP-Cre;Smarcb1 flox/flox mice present loss of SMARCB1 nuclear staining ( white arrows ), but no tumorlets or increased Ki-67 immunopositive staining. Tumorlets in DRGs of mGFAP-Cre;Smarcb1 flox/flox ;Nf2 flox/flox mice show loss of both SMARCB1 and merlin ( white and black arrows ), and tumorlets in DRGs of mGFAP-Cre;Nf2 flox/flox mice show loss of merlin only ( black arrows ). Both tumorlets from mGFAP-Cre;Smarcb1 flox/flox ;Nf2 flox/flox and mGFAP-Cre;Nf2 flox/flox mice show strong positive staining for FABP7 and GFAP ( black arrows ). Tumorlets from these both genotypes are S100 positive ( black arrows ) or negative ( white arrows ). Ki-67 positive staining is found in tumorlets of both mGFAP-Cre;Smarcb1 flox/flox ;Nf2 flox/flox and mGFAP-Cre;Nf2 flox/flox mice ( arrowhead ). Inset scale bar : 15 µm Full size image Patients with germline mutations of the SMARCB1 gene are predisposed to develop RTs or schwannomas, two tumor types with dramatically different clinical features. However, the presence of aggressive PNS tumors with rhabdoid features suggests a link between the development of RTs and schwannomas [20] . We used the P0-CreC mouse line, known to express the Cre recombinase in NCCs, to target the precursors of the SC lineage and the schwannoma cells of origin [42] (Fig. 7 ). The early onset and high penetrance of RTs in P0-CreC;Smarcb1 flox/flox mice demonstrated that loss of Smarcb1 in early NC (E9.5) is necessary for RT tumorigenesis (Fig. 7 ). This result is consistent with the high penetrance of AT/RTs in Rosa26-CreERT2;Smarcb1 flox/flox mice injected with tamoxifen between E6 and E10 [30] . Although the Rosa26-CreERT2 model doesn’t target Smarcb1 deletion in a specific cell type, expression profiling suggests that the cell of origin could be ectomesenchyme, a cephalic NCC-derived mesoderm or neural progenitors depending of the tumor subtype [30] . Inactivation of Smarcb1 at later stages of SC development failed to initiate tumorigenesis in DHH-Cre;Smarcb1 flox/flox and mGFAP-Cre;Smarcb1 flox/flox mice suggesting that Smarcb1 loss is not tumorigenic in the peripheral SC lineage or in the brain glial cells when the deletion is induced after E12.5 or E13.5, respectively (Fig. 7 ); or that the neurological deficits were lethal before the mice developed tumors. This result is consistent with other studies demonstrating that single loss of Smarcb1 in hGFAP -positive neural precursors is not tumorigenic [44] , [56] and that additional loss of Trp53 is required to induce AT/RT development in hGFAP-Cre;Smarcb1 flox/flox ;Trp53 flox/flox mice [44] . The use of different Cre drivers allowed us to narrow down the temporal window during which Smarcb1 loss is tumorigenic. The existence of a specific developmental time window could also explain the presence of RTs and schwannomatosis within a family sharing the same SMARCB1 mutation [15] , [16] , [17] . The neurological deficits developed by DHH-CreC;Smarcb1 flox/flox , mGFAP-Cre;Smarcb1 flox/flox and mGFAP-Cre;Smarcb1 del/flox mice with late Smarcb1 inactivation also point to a role of Smarcb1 in nervous system development, which could underlie the neurological deficits found in the SMARCB1 -related human Coffin–Siris syndrome [61] . Fig. 7 Proposed model of schwannoma versus RT initiation in the NC-derived SC lineage. Schematic illustration of the different combinations of mouse genotypes modeling different steps of the human 4-hit/3-step mechanism sequence and corresponding tumor phenotypes. a Smarcb1 loss in early NC results in RT development in P0-CreC;Smarcb1 flox/flox mice, but is not tumorigenic when occurring at later SC developmental stages ( DHH-Cre;Smarcb1 flox/flox and mGFAP-Cre;Smarcb1 flox/flox mice). Thus, loss of Smarcb1 does not contribute to schwannoma development in mGFAP-Cre;Smarcb1 flox/flox ;Nf2 flox/flox mice where Nf2 loss in the SC lineage is sufficient for tumor initiation, as b in mGFAP-Cre;Nf2 flox/flox mice. *germline Smarcb1 allele inactivation Full size image The fact that most of the tumors were found in the head of P0-CreC;Smarcb1 flox/flox mice is consistent with early Cre expression under the control of the P0 promoter in cranial NCCs and the prominent expression of Smarcb1 between E8 and E11.5 during the embryonic development of the headfolds, neural folds and first brachial arch [34] . P0 was originally identified as a SC-specific myelin structural protein, but was more recently found expressed by migrating NCCs in the head of E10.5 mouse embryos [62] , as well as in the otic placode and migrating cranial NCCs of E10 rat embryos. After E11, P0 can be detected in the ophthalmic and submandibular branches of the trigeminal nerves, within the trigeminal ganglion and in the developing acoustic/facial nerves of rat embryos. The P0-CreC transgene used in this study is expressed in the head of mouse embryos as early as E9.5 [25] . The presence of craniofacial abnormalities confirms the early inactivation of Smarcb1 in the cranial NC, which is at the origin of multiple head structures such as bones and cartilages, SCs, olfactory ensheathing cells and meninges. The high frequency of tumors originating in the olfactory nerve is likely due to the fact that olfactory ensheathing cells, as opposed to the non-myelinating SCs of the trunk, do not down regulate P0 expression. Therefore, the promoter driving the Cre recombinase is continuously activated in the olfactory ensheathing cells of P0-CreC;Smarcb1 flox/flox mice. Activity of the P0-Cre transgene has also been demonstrated in the enteric ganglia [63] , thus explaining the presence of bloated intestine resulting from defects of the enteric nervous system, which is derived from vagal and sacral NCCs. The presence of RTs in the subarachnoid space, in the rostral part of the cortex is consistent with the hypothesis that these tumors developed from the cranial NC-derived meningeal progenitor cells [39] . Although in patients AT/RTs are predominantly infratentorial, they can also develop in the supratentorial region of the brain with frequent connection to the ventricles [64] . Human RTs have also been described in the meninges [65] . The early NC origin of P0-CreC;Smarcb1 flox/flox RTs is also supported by expression of early NC specification markers and SWI-SNF subunits characteristic of undifferentiated cells. Altogether, these results strongly support the hypothesis that both PNS and meningeal RTs originate from NCCs. Tumors found in P0-CreC;Smarcb1 flox/flox mice displayed histological features strikingly similar to human RTs, including aggressive growth, characteristic histological patterns and presence of rhabdoid cells [40] . The anatomical locations of RTs in P0-CreC;Smarcb1 flox/flox mice have all been described in human RT patients: optic [22] , oculomotor [66] , trigeminal [21] , vestibulochochlear [23] nerves, eye [67] , nasal cavities [68] , meninges [65] and spine [69] . About 60% of P0-CreC;Smarcb1 flox/flox mice displayed multiple tumors at the time of dissection, which is consistent with the occurrence of synchronous RTs in some patients with SMARCB1 mutations [66] . Finally, molecular profiling showed that P0-CreC;Smarcb1 flox/flox RTs represented the full spectrum of human AT/RT molecular subtypes [43] . Although in mGFAP-Cre;Smarcb1 flox/flox ;Nf2 flox/flox mice loss of Smarcb1 and Nf2 is synchronous and not sequential as postulated by the 4-hit/3-step model, this is the first tumor model reproducing the genetic profile of schwannomatosis-schwannomas with concomitant loss of both Smarcb1 and Nf2 genes, with schwannoma and no RT development (Fig. 7 ). The mGFAP-Cre;Smarcb1 flox/flox ;Nf2 flox/flox mouse model demonstrates that biallelic loss of Smarcb1 loss is dispensable and Nf2 loss is necessary for schwannoma development [41] , as in mGFAP-Cre;Nf2 flox/flox mice. This is consistent with the presence of NF2 somatic mutations in the vast majority of schwannomas in schwannomatosis patients [10] , [11] . Similar to schwannomatosis patients, loss of both Smarcb1 and Nf2 does not increase the malignancy of mGFAP-Cre;Smarcb1 flox/flox ;Nf2 flox/flox tumors compared to mGFAP-Cre;Nf2 flox/flox tumors with single Nf2 loss. In contrast to NF2, schwannomas in schwannomatosis patients are typically distinctly painful, rather than manifesting with localized neurologic deficits [2] . Thus, Smarcb1 inactivation could be responsible for the pain phenotype, as suggested by a report showing that loss of Smarcb1 in adult mouse SC induces the expression of a secreted factor that in turn increases TRPV1 expression and thermal sensitivity [70] . In conclusion, we found that biallelic inactivation of Smarcb1 in the NC leads to the development of PNS and meningeal RTs, thus identifying the cell of origin for these RT subsets in an early NC population. We also defined an early spatio-temporal window during which Smarcb1 loss results in malignant tumor formation and showed that biallelic Nf2 loss is necessary and Smarcb1 loss is dispensable for schwannoma formation. This mouse model developing schwannomas with the same underlying gene mutations found in schwannomatosis patients will prove invaluable for the study of other schwannomatosis-associated phenotypes, such as neuropathic pain. Mice and genotyping All mouse strains were maintained on FVB/N genetic background. Mice were monitored twice a week for 24 months or until a tumor or evidence of a tumor (paralysis, swelling, lethargy) was observed. All animal care and experimentation were performed with the approval of the Institutional Animal Care and Use Committees under protocol number HE1175-10-02. Smarcb1 del/+ mice were obtained by breeding mGFAP-Cre;Smarcb1 flox/+ males (expressing Cre in the germline, http://www.jax.org/strain/024098 ) with wild-type FVB females. mGFAP-Cre;Smarcb1 del/flox mice were obtained by breeding mGFAP-Cre;Smarcb1 flox/+ males with Smarcb1 flox/flox females. Mice were genotyped by PCR amplification of DNA extracted from tail biopsies using the primers cre-s1 (5′-ACA TGT TCA GGG ATC GCC AG-3′) and cre-a1 (5′-TAA CCA GTG AAA CAG CAT TGC-3′) for the Cre transgene, 407Fbis (5′-GGA AAA TCT AGA AAG CAC AAA TGA-3′) and 408R (5′-TGT AGT CTA GGC TGG GTG TG-3′) for the Smarcb1 WT and Smarcb1 flox alleles, 407Fbis and 416rbis (5′-CCT GGG GCA GCT CTC TAC A-3′) for the Smarcb1 del allele, NF2Flox2-S (5′-CTT CCC AGA CAA GCA GGG TTC-3′) and NF2Flox2-A (5′-GAA GGC AGC TTC CTT AAG TC-3′) for the Nf2 WT and Nf2 flox alleles and Z1 (5′-GCG TTA CCC AAC TTA ATC G-3′) and Z2 (5′-TGT GAG CGA GTA ACA ACC-3′) for the AZCL transgene. Magnetic resonance imaging Mice were anesthetized with isoflurane throughout the imaging procedure. Mice were inserted in the prone position into a small animal MRI scanner (PharmaScan 300; Bruker BioSpin Division, Billerica, MA, USA) 7 Tesla magnet using the 19-mm inner diameter transmit receive coil. ParaVision 4.0 scanner software (BRUKER BioSpin MRI GmbH, Ettlingen, Germany) was set to use Rapid Acquisition with Relaxation Enhancement (RARE) spin echo sequence for fast T2-weighted imaging (TE 50, TR 3000, RARE Factor 8) with a 256 × 256 in-plane matrix and a 2.56-cm field of view. After scanning, if needed, mice were gently warmed on a thermostatically controlled heating pad until awake enough to be returned to their home cage. MRI images were reconstructed at native resolution and analyzed with OsiriX (Open-Source Software for Navigating in Multidimensional DICOM Images) image analysis software packages. H&E staining, immunohistochemistry, X-gal staining and cell counting Hematoxylin and eosin staining was performed on 3.5-µm-thick sections prepared from paraffin blocks of formalin-fixed tissues. Immunohistochemistry was performed on 9 P0-CreC;Smarcb1 flox/flox representative tumors (3 tumors per histological pattern) and 7 representative schwannomas from P0-CreC;Nf2 flox/flox mice (Fig. 3 and Supplementary Table 1 ). A standard protocol was used with primary antibodies incubated 1 h at room temperature: cytokeratin (1/500, Dako, M3515), FABP7 (1/1000, Abcam, ab32423), GFAP (1/3000, Dako, Z0334), Ki-67 (1/1000, BD Pharmingen, 556003), merlin (1/400, Cell Signaling Technology, #6995), neurofilament triplet proteins (1/500, Enzo Life Sciences, BML-NA1223), PGDS (1/1000, Santa Cruz Biotechnology, sc-14826), S100 (1/10000, Dako, Z0311), SMA (1/200, BioCare Medical, CME 305), SMARCB1 (1/200, BD Transduction Laboratories, 612110), vimentin (1/200, Cell Signaling Technology, #5741). Biotinylated secondary anti-rabbit, anti-mouse (Vector Laboratories, Burlingame, CA) or anti-goat (Dako) IgG antibodies were incubated 30 min at room temperature. Immunoreactivity was semi-quantitatively scored based on the percentage of positive tumor cells (few, foci or majority of positive cells) and the intensity of staining (weak, moderate or strong). To assess cell proliferation, bromodeoxyuridine (50 mg/kg body weight) was administrated 4 h before dissection of the tissues. Incorporation of BrdU was then revealed by immunohistochemistry with BrdU antibody (Fitzgerald Industries International, 20-BS17) and secondary anti-sheep antibody (Jackson ImmunoResearch Laboratories, West Grove, PA). For X-gal staining, tissues were frozen in OCT compound (Tissue-Tek, 4583) on dry ice. Frozen sections of 10 µm were fixed in 2% formaldehyde and 0.2% glutaraldehyde in 1X PBS for 10 min at room temperature. Fixed tissues were washed three times in 1X PBS, and incubated overnight at 37 °C in the staining solution (5 mM K 3 [Fe(CN) 6 ], 5 mM K 4 [Fe(CN) 6 ], 2 mM MgCl 2 and 2 mg/ml X-gal in PBS). After staining, tissues were washed twice in 1× PBS and counterstained with Nuclear Fast Red for 1–2 min. For DRG cell count, 5–12 DRGs of the cervical and/or thoracic spine were selected from 3–5 mice per genotype using a light microscope Axio Imager M1 (Zeiss). The region of interest (ROI) containing ganglion cells was manually demarcated on captured images of 20× magnification fields. The Axiovision software was used to determine the surface and the cells count in the ROI. All histopathological analysis was performed in blind under the guidance of an experienced pathologist. PCR PCR amplification was performed on DNA extracted from multiple tissues using the primers cre-s1 and cre-a1 for the Cre transgene, 407Fbis and 408R for the Smarcb1 WT and Smarcb1 flox alleles, 407Fbis, 408R, and 416R (5′-GCC ACC AGC CAG ATG TCA TAC-3′) for the Smarcb1 flox and Smarcb1 del alleles in the tumors, Ini1DelAf (5′-AAG CAC AAA TGA GAG AAA ACG TA-3′) and Ini1DelBr (5′-TGC CAC CAG CCA GAT GTC A-3′) with Hotmaster Taq DNA polymerase for the Smarcb1 del allele in the PCR for all the tissues. RNA-Seq and bioinformatics RNA was isolated using the RiboPure kit (Life Technologies) according to manufacturer’s instructions. RNA Libraries were prepared using the TruSeq Stranded library preparation kit (Illumina) RNA after RiboZero treatment for removal of ribosomal RNAs. After library preparation, amplified double-stranded cDNA was fragmented into 125 bp (Covaris-S2, Woburn, MA) DNA fragments, which were (200 ng) end-repaired to generate blunt ends with 5′- phosphates and 3′- hydroxyls and adapters ligated. The purified cDNA library products were evaluated using the Agilent Bioanalyzer (Santa Rosa, CA) and diluted to 10 nM for cluster generation in situ on the HiSeq paired-end flow cell using the CBot automated cluster generation system. All samples were multiplexed into a single pool in order to avoid batch effects and sequenced using an Illumina HiSeq 4000 sequencer (Illumina, San Diego, CA) yielding between 52 and 90 million reads per sample. Quality control was performed on base qualities and nucleotide composition of sequences. 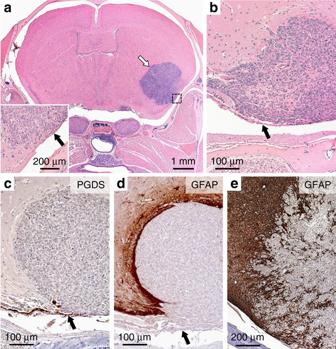Fig. 2 P0-CreC;Smarcb1flox/floxmice develop RTs in the meninges.aSupratentorial tumors (white arrow) were found predominantly located in the subarachnoid space (black arrow, inset) with extension into the brain parenchyma.Insetrepresents a higher magnification of thedashed square area.bDetail of a tumor originating from the meninges. Thearrowshows the arachnoid cell layer.cNo PGDS staining was found in the tumor as opposed to the arachnoid cell layer (arrow).d,eThe GFAP staining demonstrated the different degree (d, non-invasive;e, irregular tumor brain interface consistent with infiltration) of invasiveness of the tumors in the brain tissue Alignment to the M. musculus (mm10) refSeq (refFlat) reference gene annotation was performed using the STAR spliced read aligner with default parameters. Additional QC was performed after the alignment to examine: the level of mismatch rate, mapping rate to the whole genome, repeats, chromosomes, key transcriptomic regions (exons, introns, UTRs, genes), insert sizes, AT/GC dropout, transcript coverage and GC bias. Between 80 and 85% (average 83%) of the reads mapped uniquely to the mouse genome and only uniquely mapped reads were used for subsequent analyses. Total counts of read-fragments aligned to candidate gene regions were derived using HTSeq program (version 0.6.0, www.huber.embl.de/users/anders/HTSeq/doc/overview.html ) with mouse mm10 refSeq (refFlat table) as a reference and used as a basis for the quantification of gene expression. Microarray data from Johann et al. [43] (GSE70678), Han et al. [30] (GSE64019) and Ng et al. 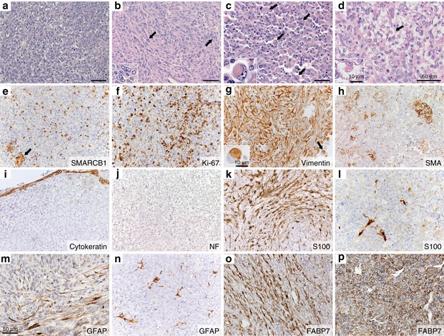Fig. 3 RTs ofP0-CreC;Smarcb1flox/floxmice display typical histological and immunohistochemical staining features of human RTs.aTumor presenting a primitive neuroectodermal pattern.bTumor with mesenchymal pattern characterized by spindle-shaped cell component and nuclei showing vesicular chromatin staining pattern with prominent nucleoli (arrows and inset).cNest of classic rhabdoid cells with eccentrically placed nuclei, vesicular chromatic staining and eosinophilic cytoplasm inclusion (arrows and inset).dTumor demonstrating vacuolar cytoplasmic degeneration pattern (arrow and inset).eSMARCB1 staining shows loss of nuclear expression in tumor cells with retained expression in infiltrating inflammatory cells and intratumoral vasculature (arrow).fKi-67 staining reveals high proliferative index.gDiffuse strong expression of vimentin in tumor tissue fromP0-CreC;Smarcb1flox/floxmice. Note the staining of the cytoplasmic inclusions in rhabdoid cells (arrow and inset).hFoci of tumors cells show positive cytoplasmic staining for SMA.i,jNo staining of cytokeratinsiand neurofilament triplet proteinsjwere found in the tumors.kStrong S100 immunoreactivity in schwannoma fromP0-CreC;Nf2flox/floxmice.lNo S100 staining is present in the tumors cells ofP0-CreC;Smarcb1flox/floxmice. Sparse positive cells are entrapped residual normal cells.mModerate GFAP staining inP0-CreC;Nf2flox/floxschwannoma.nNo GFAP staining is present in the tumors cells ofP0-CreC;Smarcb1flox/floxmice.o,pStrong expression of FABP7, an early marker of SC precursors, inP0-CreC;Nf2flox/floxoandP0-CreC;Smarcb1flox/floxptumors.Scale bars: 50 µm for main pictures and 10 µm forinsets [44] (GSE68627) was downloaded from GEO and normalized using the robust multiarray method (RMA). Gene symbols were used to match human and mouse transcripts and merge expression datasets after averaging multiple probes querying the same gene. Batch effects were corrected using ComBat and overall quantile normalization was performed across data sets. Hierarchical clustering of the top most variable genes (as ranked by s.d.) 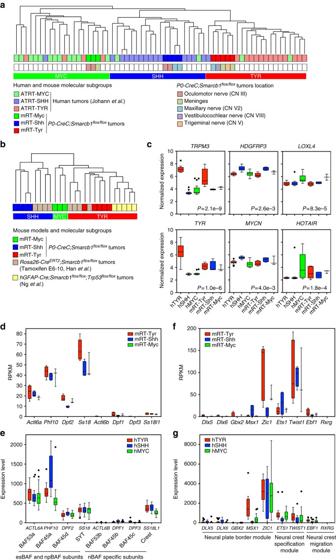Fig. 4 Molecular profiling of RTs fromP0-CreC;Smarcb1flox/floxmice.aUnsupervised hierarchical clustering of gene expression profiles from 12P0-CreC;Smarcb1flox/floxmouse tumors and 49 human AT/RTs43using the 5,000 most variable transcripts. TheP0-CreC;Smarcb1flox/floxtumors distributed among the three human AT/RT molecular subgroups. Information about tumor molecular subgroups and anatomical location is displayed in the lower bars.bUnsupervised hierarchical clustering of gene expression profiles from 12P0-CreC;Smarcb1flox/floxmouse tumors, eight tumors from the tamoxifen inducibleRosa26-CreERT2;Smarcb1flox/floxmouse model30and five tumors from thehGFAP-Cre;Smarcb1flox/flox;Trp53flox/floxmouse model44using the 5,000 most differentially expressed genes. Information about tumor molecular subgroups is displayed in the lower bars.cNormalized expression level of representative genes for both of the three human AT/RT molecular subgroups: hTYR (n= 16), hSHH (n= 16), and hMYC (n= 17) and the threeP0-CreC;Smarcb1flox/floxRT molecular subgroups: mRT-Tyr (n= 5), mRT-Shh (n= 4) and mRT-Myc (n= 3). On the basis of the cluster analysis in (a), we respectively named hMYC, hSHH and hTYR the three tumor subgroups including human tumors from the MYC, SHH and TYR molecular subgroups43. TheP-value indicates the statistical significance of gene enrichment within their respective WGCNA module for each respective molecular subgroup.d–gGene expression levels of specific SWI/SNF complex subunits (d,e) and NC developmental markers (f,g) in the three molecular subgroups ofP0-CreC;Smarcb1flox/floxRTs (d,f) and human AT/RTs (e,g).d,fRNA-Seq data are expressed in RPKM (Reads Per Kilobase of transcript per Million mapped reads).e,ggraphs of microarray gene-expression intensity from dataset GSE70678.c–gRNA-Seq and microarray gene expression levels are shown using Tukey boxplots: thecentral linesrepresent the median,boxes(interquartile range or IQR) represent 50% of data ranging from the 25 to 75% quantile,whiskersrepresent extremes up to 1.5-fold box size,circlesshow outliers was performed using the plotDendroAndColors function from the WGCNA package. Weighted Gene Co-expression Network Analysis (WGCNA) was conducted using the R package. Briefly, correlation coefficients were constructed between expression levels of genes, and a connectivity measure (topological overlap, TO) was calculated for each gene by summing the connection strength with other genes. Genes were then clustered based on their TO, and groups of co-expressed genes (modules) were identified. Each module was assigned a color, and the first principal component (eigengene) of a module was extracted from the module and considered to be representative of the gene expression profiles in a module. The phenotypic trait of interest is then regressed on the eigengene to examine whether there was a significant relationship between the module and the trait. The optimal number of clusters was determined using the non-negative matrix factorization (NMF) method with the NMF R package, based on the top 5000 most variable genes with standard NMF algorithm method (brunet) performed on 10 runs. The optimal numbers of clusters have been defined based on the maximum cophenetic correlation score. Quantitative RT-PCR Reverse transcription was performed with 1 µg of the same RNA samples used for RNA-Seq and the SuperScript IV VILO Master Mix (Life Technologies) following the manufacturer’s instructions. Gene expression levels were assessed by quantitative PCR using a QuantStudio 3 real-time PCR system (Applied Biosystems) and TaqMan gene expression assays: Smarcb1 (Mm00448776_m1), Ezh2 (Mm00468464_m1) and Hprt (Mm00446968_m1, Life Technologies). Relative expression was determined using the 2 −∆∆Ct method with Hprt expression as reference and normalized to a brain control sample. 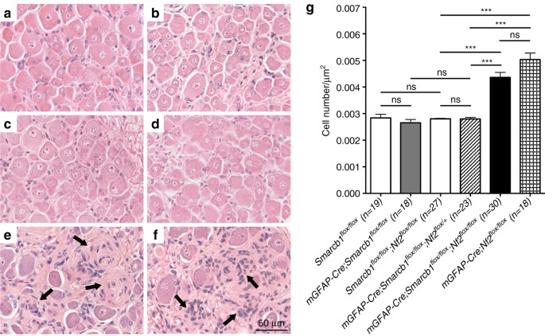Fig. 5 Biallelic loss ofNf2is necessary to induce schwannoma formation.a,bNo difference in cellularity of DRGs frommGFAP-Cre;Smarcb1flox/floxmice (b) compared withSmarcb1flox/floxcontrol mice (a).c–fThe loss of one additionalNf2allele inmGFAP-Cre;Smarcb1flox/flox;Nf2flox/+mice does not impair the DRG cellularity (d) compared tomGFAP-Cre;Smarcb1flox/floxmice (b) orSmarcb1flox/flox;Nf2flox/floxcontrol mice (c). The biallelic lossNf2induced the formation of schwannoma tumorlets inmGFAP-Cre;Smarcb1flox/flox;Nf2flox/floxmice (e), similar tomGFAP-Cre;Nf2flox/floxmice (f).gNumber of cells per DRG surface for each genotype. Data are represented as mean ± s.e.m.;nis the number of DRG analyzed per genotype, ns (not significant), ***(P< 0.001), two-tailed unpaired Student’st-test Western blot Tissues were snap-frozen in liquid nitrogen and stored at −80 °C. Pulverized frozen tumor samples were lysed in radioimmunoprecipitation assay (RIPA) buffer and the total proteins were extracted, separated, and transferred using standard procedures. Antibodies were purchased from BD Transduction Laboratories: SMARCB1 (1/500, 612110); Cell Signaling Technology: Akt (1/2000, #9272), P-Akt (Ser473) (1/2000, #4060), CDK4 (1/2000, #2906), CDK6 (1/2000, #3136), Cyclin D1 (1/3000, #2926), merlin (1/1000, #6995), p27 (1/1000, #2552), P-Rb (1/1000, #8516), S6 (1/1000, #2317), P-S6 (Ser 235/236) (1/4000, #4858), 4E-BP1 (1/2000, #9452); Novus Biologicals: GAPDH (1/5000, NB300-221), PTCH1 (1/1000, MAB41051), RB1 (1/50, NB120-3077), SHH (1/500, AF464); R&D Systems: GLI-1 (1/1000, AF3455); Santa Cruz Biotechnology: p16 (1/3000, sc-1207) and Thermo Scientific: p21 WAF1 (1/1000, MS-387-P0). All uncropped scans of western blots are provided in Supplementary Fig. 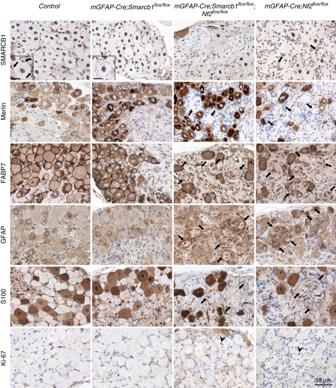Fig. 6 Histological characterization of DRGs and schwannoma tumorlets in control,mGFAP-Cre;Smarcb1flox/flox,mGFAP-Cre;Smarcb1flox/flox;Nf2flox/flox, andmGFAP-Cre;Nf2flox/floxmice. DRGs frommGFAP-Cre;Smarcb1flox/floxmice present loss of SMARCB1 nuclear staining (white arrows), but no tumorlets or increased Ki-67 immunopositive staining. Tumorlets in DRGs ofmGFAP-Cre;Smarcb1flox/flox;Nf2flox/floxmice show loss of both SMARCB1 and merlin (white and black arrows), and tumorlets in DRGs ofmGFAP-Cre;Nf2flox/floxmice show loss of merlin only (black arrows). Both tumorlets frommGFAP-Cre;Smarcb1flox/flox;Nf2flox/floxandmGFAP-Cre;Nf2flox/floxmice show strong positive staining for FABP7 and GFAP (black arrows). Tumorlets from these both genotypes are S100 positive (black arrows) or negative (white arrows). Ki-67 positive staining is found in tumorlets of bothmGFAP-Cre;Smarcb1flox/flox;Nf2flox/floxandmGFAP-Cre;Nf2flox/floxmice (arrowhead).Inset scale bar: 15 µm 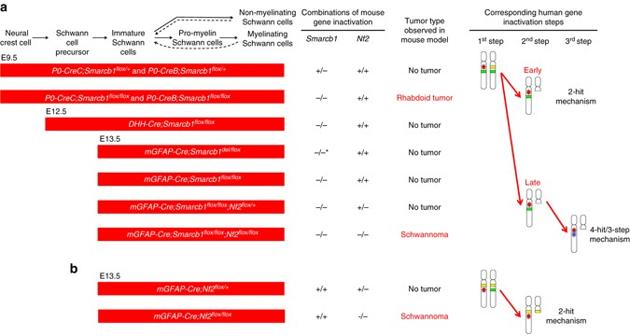Fig. 7 Proposed model of schwannoma versus RT initiation in the NC-derived SC lineage. Schematic illustration of the different combinations of mouse genotypes modeling different steps of the human 4-hit/3-step mechanism sequence and corresponding tumor phenotypes.aSmarcb1loss in early NC results in RT development inP0-CreC;Smarcb1flox/floxmice, but is not tumorigenic when occurring at later SC developmental stages (DHH-Cre;Smarcb1flox/floxandmGFAP-Cre;Smarcb1flox/floxmice). Thus, loss ofSmarcb1does not contribute to schwannoma development inmGFAP-Cre;Smarcb1flox/flox;Nf2flox/floxmice whereNf2loss in the SC lineage is sufficient for tumor initiation, asbinmGFAP-Cre;Nf2flox/floxmice. *germlineSmarcb1allele inactivation 7 . Statistical analysis GraphPad Prism software version 5.0 (GraphPad Software, San Diego, CA) was used to perform statistical analysis and construct Kaplan–Meier survival curves. Mendelian birth incidence of mouse genotypes was examined using chi-square test. Differences in survival of mouse genotypes were analyzed by log-rank Mantel–Cox test. Two-tailed Student’s unpaired t -test was used to determine significance between groups unless otherwise indicated. The variance between the groups was not significantly different (F test). A P value of < 0.05 was considered statistically significant. Results of the significance tests are reported as follow: ns (non significant), *( P < 0.05), **( P < 0.01) and ***( P < 0.001). Error bars represent s.e.m. Data availability The RNA-Sequencing data presented in this study have been deposited in NCBI Gene Expression Omnibus with the accession number GSE94082. All other data supporting the findings of this study are available in Supplementary Information Files and from the corresponding author upon reasonable request.